A new class of Solvent-in-Salt electrolyte for high-energy rechargeable metallic lithium batteries Liquid electrolyte plays a key role in commercial lithium-ion batteries to allow conduction of lithium-ion between cathode and anode. Traditionally, taking into account the ionic conductivity, viscosity and dissolubility of lithium salt, the salt concentration in liquid electrolytes is typically less than 1.2 mol l −1 . Here we show a new class of ‘Solvent-in-Salt’ electrolyte with ultrahigh salt concentration and high lithium-ion transference number (0.73), in which salt holds a dominant position in the lithium-ion transport system. It remarkably enhances cyclic and safety performance of next-generation high-energy rechargeable lithium batteries via an effective suppression of lithium dendrite growth and shape change in the metallic lithium anode. Moreover, when used in lithium–sulphur battery, the advantage of this electrolyte is further demonstrated that lithium polysulphide dissolution is inhibited, thus overcoming one of today’s most challenging technological hurdles, the ‘polysulphide shuttle phenomenon’. Consequently, a coulombic efficiency nearing 100% and long cycling stability are achieved. Lithium-based batteries as highly efficient energy storage devices have long been considered as promising power supply for various electric vehicles and smart grid storage systems [1] , [2] , [3] , [4] . However, presently available lithium-ion technology cannot satisfy the increasing demand for energy density. Metallic lithium batteries exhibit the highest theoretical energy densities among the secondary batteries [5] . Among many possible systems, lithium–sulphur (Li–S) and lithium–oxygen (Li–O 2 ) batteries are quite attractive as candidates for next-generation high-energy density batteries [5] , [6] , [7] , [8] , [9] , [10] , [11] , [12] , [13] , [14] , [15] , [16] , [17] , [18] , [19] , [20] , [21] , [22] . However, the application of metallic lithium anode suffers from inevitable formation of lithium dendrites, which are caused by uneven current distributions at the metal–electrolyte interface during cycling. The formation of lithium dendrites will lead to poor cyclic performance and increase the probability of internal short circuit, resulting in safety issues. Thus, great effort has been paid to suppress the formation of lithium dendrites and reduce metallic lithium corrosion in liquid electrolytes [23] . For instance, the use of solid polymer or inorganic electrolytes could potentially suppress the formation of the lithium dendrites. However, for solid-state electrolytes, the kinetic properties are limited, due to both low conductivity at room temperature and high interfacial resistance [24] , [25] , [26] , [27] , [28] . Recently, a breakthrough has been achieved in inorganic sulphide-based electrolytes with quite high room temperature conductivity of 10 −2 S cm −1 (ref. 29 ). The application of Li 2 S–P 2 S 5 glass–ceramic electrolyte in Li–S batteries has been demonstrated [30] , [31] , [32] . To reduce the interfacial resistance, 30wt.% solid electrolyte and 35wt.% acetylene black were required to add into sulphur electrode [32] . This leads to a decrease in energy density of Li–S batteries. It seems that the strategy of physical mixing of active phase and solid electrolyte still suffers from point-to-point contact [30] , [31] , [32] , not like a complete surface-to-surface wetting effect as liquid electrolyte. Here we report a new class of non-aqueous liquid ‘Solvent-in-Salt’ electrolytes and apply them in Li–S batteries. It is demonstrated that the use of ‘Solvent-in-Salt’ electrolyte inhibits the dissolution of lithium polysulphide, effectively protects metallic lithium anodes against the formation of lithium dendrites and results in high lithium cycling efficiency, thus enhancing electrochemical performance. The concept of ‘Solvent-in-Salt’ electrolyte In 1993, Angell et al . [33] proposed the innovative concept of ‘Polymer-in-Salt’ by reversing the ratio of solid polymer solvent to salt, in which glass transition ( T g ) was low enough to remain rubbery at room temperature to preserve good conductivity and high electrochemical stability. However, in practice the T g remained above ambient temperature and/or the system would crystallize. For conventional non-aqueous organic electrolytes, the salt concentration is usually limited in a range of 1–2 mol l −1 , which is a trade-off among ionic conductivity, viscosity and salt solubility. Thus, most of the studies focus on the region C of Fig. 1 , in which there is much less salt than solvent. There are few reports of research in the A (yellow) or D (green) regions of Fig. 1 , in which either the weight or volume ratio of salt-to-solvent exceeds 1.0 (refs 34 , 35 , 36 , 37 ). As a matter of fact, by choosing proper salt and solvent, we can move an electrolyte into those regions (A, B and D) and also obtain some unexpected properties. To distinguish from traditional electrolytes, this new class of electrolyte is denoted by ‘Solvent-in-Salt’ (SIS). A similar system of hydrated molten salt composed of KNO 3 and Ca(NO 3 ) 2 ·4H 2 O, in which the water content is insufficient to satisfy more than a first coordination sheath for the cation that was reported in 1965 by Angell [38] , [39] . This kind of hydrated molten salts was usually used in heat storage but not called SIS. 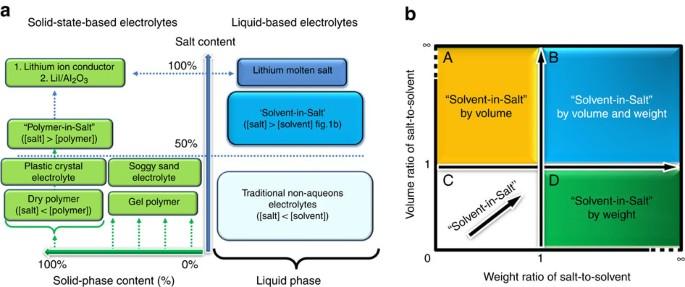Figure 1: A general concept for Solvent-in-Salt electrolyte. (a) The overview of the available electrolytes58,59,60. (b) The distribution map of non-aqueous liquid electrolytes with the weight and volume ratios of salt-to-solvent. A, B and D regions are Solvent-in-Salt electrolyte, in which the ratio of salt-to-solvent is over 1.0 by volume or weight. C region is [solvent]>[salt] by weight and volume. Figure 1: A general concept for Solvent-in-Salt electrolyte. ( a ) The overview of the available electrolytes [58] , [59] , [60] . ( b ) The distribution map of non-aqueous liquid electrolytes with the weight and volume ratios of salt-to-solvent. A, B and D regions are Solvent-in-Salt electrolyte, in which the ratio of salt-to-solvent is over 1.0 by volume or weight. C region is [solvent]>[salt] by weight and volume. Full size image The physicochemical properties of ‘Solvent-in-Salt’ For the following discussion, we select an electrolyte system containing Li[CF 3 SO 2 ) 2 N] (LiTFSI), one of the lowest lattice energy salts and 1,3-dioxolane (DOL): dimethoxyethane (DME) (1:1 by volume) as solvent, resulting in what we show as one of the most promising electrolytes for Li–S batteries. The physicochemical properties of this electrolyte with different ratios of salt-to-solvent are illustrated in Fig. 2 . When the mole amount of salt reaches 4 mol in 1-l solvent, the electrolyte enters the D region of SIS by weight, and beyond 5 mol salt in 1-l solvent, the salt begins to have a dominant role in either weight or volume ratio ( Fig. 2a ). Arrhenius plots of the ionic conductivity of the electrolytes with different salt concentrations in a temperature range of −20 to 60 °C are shown in Fig. 2b and exhibit the typical curvature of the Vogel–Tammann–Fulcher (VTF) equation ( Supplementary Fig. S1 ). It can be seen that the ionic conductivity decreases with increasing salt concentration. The conductivity drops slowly in the high temperature region (20–60 °C) but rapidly at a low-temperature region (−20 to 20 °C), resulting from a rise in T g . For a given electrolyte with fixed salt and solvent, ionic conductivity depends on both viscosity and lithium-ion mobility. When increasing salt concentration, more and more Li–ether complex pairs form due to incomplete solvation shell and the viscosity at room temperature increases markedly in the SIS region ( Fig. 2c and Supplementary Fig. S2 ). At the same time, the lithium-ion transference number of SIS-7# electrolyte increases to an unexpected high value ( t Li + =0.73, t Li + = σ Li + /( σ Li + + σ TFSI - )) (see Fig. 2c and Supplementary Fig. S3 ), which is much higher than that of traditional salt-in-solvent electrolytes (0.2–0.4). The conductivity of specific ion i is proportional to the concentration of mobile ion ( c i ) and its mobility ( μ i ) ( σ i =nc i μ i ). The mobility of an ion is determined by the viscosity ( η ) of the medium and radius of mobile ion ( μ i =1/6πηr i ) (ref. 23 ). In low-salt concentration electrolytes, lithium ions are coordinated with ether oxygen and form a large solvation shell compared with anions, leading to relatively lower mobility of solvated Li + cations. In the SIS system, it is plausible that the number of solvated Li + cations is decreased and large anion (TFSI − ) could be more seriously dragged than the small unsolvated cation (Li + ) in this high viscosity system. Nevertheless, SIS-7# even with a high viscosity of 72 cP retains a conductivity of 0.814 mS cm −1 at room temperature, which remains superior to that of all-solid-state dry polymer or most of the inorganic electrolytes, and especially, could form better interfacial contacts. 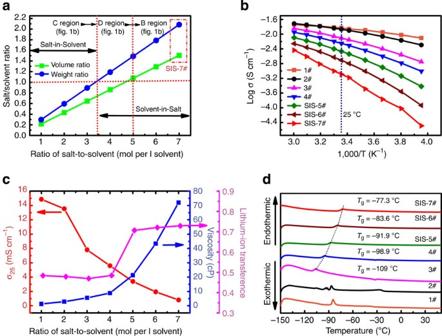Figure 2: Physicochemical properties of Solvent-in-Salt electrolytes. (a) Weight and volume ratio of salt-to-solvent with different ratios of LiTFSI to DOL:DME (1:1 by volume). (b) Arrhenius plots of the ionic conductivity as a function of 1,000/T for electrolytes with different ratios of LiTFSI to solvent, (1#: 1 mol per l solvent, 2#: 2 mol per l solvent, 3#: 3 mol l solvent, 4#: 4 mol per l solvent, 5#: 5 mol per l solvent, SIS-6#: 6 mol l per solvent and SIS-7#: 7 mol l per solvent). (c) Viscosity, ionic conductivity and lithium-ion transference number at room temperature for the aforementioned different electrolytes. (d) DSC traces of the aforementioned different electrolytes. Figure 2: Physicochemical properties of Solvent-in-Salt electrolytes. ( a ) Weight and volume ratio of salt-to-solvent with different ratios of LiTFSI to DOL:DME (1:1 by volume). ( b ) Arrhenius plots of the ionic conductivity as a function of 1,000/T for electrolytes with different ratios of LiTFSI to solvent, (1#: 1 mol per l solvent, 2#: 2 mol per l solvent, 3#: 3 mol l solvent, 4#: 4 mol per l solvent, 5#: 5 mol per l solvent, SIS-6#: 6 mol l per solvent and SIS-7#: 7 mol l per solvent). ( c ) Viscosity, ionic conductivity and lithium-ion transference number at room temperature for the aforementioned different electrolytes. ( d ) DSC traces of the aforementioned different electrolytes. Full size image Differential scanning calorimeter (DSC) traces reveal distinct glass transition temperatures ( Fig. 2d ), which shows that all the electrolytes are glass-forming liquids, and their glass transition temperatures shift from low to high, with increasing ratio of salt-to-solvent. For the pure solvent mixture without salt ( Supplementary Fig. S4 ), the glass transition temperature is −138.6 °C, justifying the excellent low temperature performance for the DOL–DME-based electrolyte. In the SIS-7# electrolyte, the value of T g is –77.3 °C, which is much lower than typical ‘Polymer-in-Salt’ system ( T g >–10 °C) (ref. 33 ) and close to that traditional commercial electrolyte systems (1 mol l −1 LiPF 6 in EC–DMC, T g =–67 °C)) (ref. 40 ). The flexible hinge in the S–N–S bond of TFSI − , specific to these imide anions, explains this ‘plasticizing effect’, which is also reflected in the low viscosities of ionic liquids based on this anion. Application in Li–S batteries The power of the SIS electrolytes is demonstrated by their use in rechargeable metallic Li–S batteries. The Li–S battery using SIS-7# as electrolyte exhibits the best electrochemical performance ( Fig. 3 ). 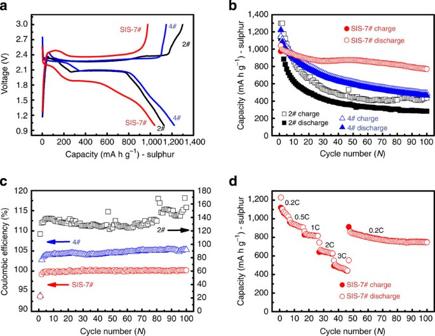Figure 3: Electrochemical performance of lithium–sulphur batteries. (a) First discharge–charge profiles of C/S electrodes in electrolytes with different ratios of LiTFSI to DOL:DME (1:1 by volume). (b) Cyclic performance. (c) Coulombic efficiency at a current rate of 0.2 C (coulombic efficiency=charge capacity/discharge capacity). (d) Rate capability with SIS-7# electrolyte. Figure 3: Electrochemical performance of lithium–sulphur batteries. ( a ) First discharge–charge profiles of C/S electrodes in electrolytes with different ratios of LiTFSI to DOL:DME (1:1 by volume). ( b ) Cyclic performance. ( c ) Coulombic efficiency at a current rate of 0.2 C (coulombic efficiency=charge capacity/discharge capacity). ( d ) Rate capability with SIS-7# electrolyte. Full size image It shows an initial specific discharge capacity of 1,041 mA h g −1 at a current rate of 0.2C (that is, 335 mA g −1 ) and maintains a reversible capacity of 770 mA h −1 g −1 with capacity retention of 74% after 100 cycles ( Fig. 3b ). More importantly, the coulombic efficiency reaches nearly 100% after the first cycle (it is 93.7% for the first cycle.) for the SIS-7# electrolyte (also see Supplementary Fig. S5 ), which is higher than previous reports in a similar system [12] , [13] , [14] , [15] , [16] , [17] , [18] , [19] , [20] , [21] , [22] , owing to effectively avoiding the polysulphide shuttle effect in the charging process ( Fig. 3c ) (ref. 41 ). In contrast, other less concentrated electrolytes exhibit an apparent coulombic efficiency greater than 100% ( Fig. 3c and Supplementary Fig. S6 ), a sign of the ‘polysulphide shuttle effect’. The only shortcoming of the use of SIS-7# is that the polarization becomes slightly larger due to relatively higher viscosity compared with traditional electrolytes with low-salt concentration ( Fig. 3a ). Yet Li–S batteries using SIS-7# electrolyte still show excellent rate capability as shown in Fig. 3d . They can achieve capacities of 1,229, 988, 864, 744 and 551 mA h g −1 of sulphur at current rates of 0.2, 0.5, 1, 2 and 3C, respectively. When the current rate returns to 0.2C, a reversible capacity of 789 mA h −1 g −1 remains. The capacity still decays after rate measurement, although the polysulphide dissolution is inhibited, which is probably related to the unstable C/S electrode. In the charge–discharge process, the electrode suffers from a large volume change by a conversion reaction between S 8 (2.07 g cm −3 ) and Li 2 S (1.66 g cm −3 ), which could result in not only the sulphur redistribution but also the structural damage of the carbon–sulphur composite. Thus, we can expect that through optimization of cathode materials, the cyclic performance will be further improved. To further prove the power of this new SIS electrolyte, the Ketjenblack without mesoporous structure was used as a support for sulphur, instead of highly ordered mesoporous carbon. It is shown that the electrochemical performance using SIS-7# electrolyte is much better than that of 2# ( Supplementary Fig. S7 ). The cycling performance is greatly improved and the coulombic efficiency is nearly 100% even with non-porous carbons as the support. This further demonstrates the extraordinary properties of this new SIS electrolyte. Currently, the electrochemical performance of Li–S batteries is directly determined by the sulphur loading in C/S composites, the adsorbability of sulphur by mesoporous carbon, the solubility of lithium polysulphide in the electrolyte and the stability of the metallic lithium anode during cycling. Actually, to date, it has seemed almost impossible to simultaneously solve all these problems via a single solution. To improve cyclic performances, one strategy is to decrease sulphur loading of the C/S composite (30–50wt.%), which not only increases electronic conductivity of C/S composites, but also enhances the absorption effect for sulphur and polysulphide, finally improving reversible storage capacity, cycling life and coulombic efficiency. However, according to our estimate of practical energy density shown in Supplementary Table S1 , it can be seen that the sulphur loading should be higher than 50wt.%; otherwise, it is difficult to achieve higher gravimetric energy density than that of advanced lithium-ion batteries. The other strategy is to add strong absorption materials such as nanosized mesoporous SiO 2 (ref. 13 ) or Mg 0.6 Ni 0.4 O (ref. 42 ), Al 2 O 3 (ref. 43 ) into a sulphur electrode, which increases the coulombic efficiency to some extent; however, the dissolution of lithium polysulphide is not completely inhibited. The third strategy is to use LiNO 3 as an effective additive to stabilize the metallic lithium anode, via an in situ formation of a protective layer on the lithium anode surface [44] , [45] . However, the protective layer can only prevent further reaction between the lithium polysulphide and the lithium anode, it is unable to inhibit the dissolution of lithium polysulphide into the electrolyte, which results in instability in terms of long cycling [16] , [46] . Finally protecting the metallic lithium anode using inorganic solid electrolyte layer prevents any soluble polysulphide reaching the lithium metal, but the brittleness of such materials prevents their use in large-surface practical systems [47] , [48] . Our Li–S batteries using SIS-7# electrolyte exhibit excellent electrochemical performance for all three aspects: (i) initial specific capacity of C/S composite with 60wt.% sulphur loading: 625 mA h g −1 , (ii) high capacity retention: 74% after 100 cycles and (iii) high coulombic efficiency: nearly 100% ( Supplementary Table S2 ). Additionally, it also shows excellent rate performance and works well in a wide temperature range even to −20 °C ( Supplementary Fig. S8 ). All those significant improvements derive from two reasons. First, the dissolution of lithium polysulphide is effectively reduced, thus avoiding lithium polysulphide shuttle phenomenon. In Li–S batteries, the soluble intermediate is mainly Li 2 S n (8≤n≤4) produced during initial discharge and final charge stages. It can be considered to be a lithium salt, and its solubility has a certain saturation degree for a given solvent. Thus, for the electrolyte with ultrahigh lithium salt concentration such as SIS-7#, the concentration is almost close to saturation, in which case the soluble intermediate (Li 2 S n ) becomes hardly soluble, as further proven in Fig. 4 . The colour of 7# (SIS-7#) is nearly unchanged after standing for 18 days. In contrast, all others show colour change from dark-brown to yellow, which is consistent with the ultraviolet-visible (UV-Vis) spectra ( Fig. 4b ). After equal proportional dilution, those three samples (2#, 4# and 7#) are obviously different in UV-Vis light absorption. Among them, the curves of 7#, 4#′ and 7#′ are nearly superimposed in the whole region, which indicates that the dissolution of lithium polysulphide is indeed inhibited in the SIS-7# electrolyte. During the review process, we noticed that a very recent work simply showed that a higher salt concentration electrolyte (but only up to 5 M) is helpful to decrease both the dissolution of lithium polysulphide and the diffusion coefficient of bulky polysulphide in the electrolyte, thus improving the coulombic efficiency [49] . Actually, the dissolution of lithium polysulphide is not totally prohibited because in this case the highest concentration used was 5 M LiTFSI in DME/DOL. 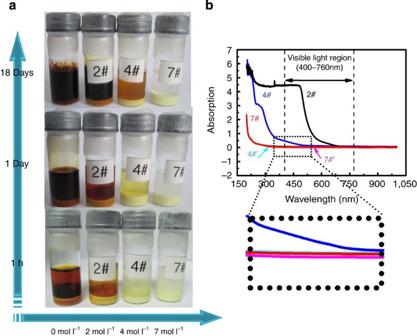Figure 4: Lithium polysulphide dissolution experiments. (a) The colour changes of four samples with different salt concentrations containing the same amount of Li2S8were recorded by digital camera along with time: 0 mol per l solvent, 2#: 2 mol per l solvent, 4#: 4 mol per l solvent, 7#: 7 mol per l solvent. (b) The ultraviolet-visible spectrophotometry. The 2#, 4# and 7# for UV-Vis measurement are the solutions from the standing samples for 18 days, which are then diluted with the corresponding electrolytes in a volume ratio of 1:7. The curves of 4#' and 7#' are the pure electrolytes of 4 mol per l solvent and 7 mol per l solvent for comparison, respectively. Figure 4: Lithium polysulphide dissolution experiments. ( a ) The colour changes of four samples with different salt concentrations containing the same amount of Li 2 S 8 were recorded by digital camera along with time: 0 mol per l solvent, 2#: 2 mol per l solvent, 4#: 4 mol per l solvent, 7#: 7 mol per l solvent. ( b ) The ultraviolet-visible spectrophotometry. The 2#, 4# and 7# for UV-Vis measurement are the solutions from the standing samples for 18 days, which are then diluted with the corresponding electrolytes in a volume ratio of 1:7. The curves of 4#' and 7#' are the pure electrolytes of 4 mol per l solvent and 7 mol per l solvent for comparison, respectively. Full size image Second, a metallic lithium anode is more stable in the SIS-7# electrolyte than in other electrolytes. Compared with other kinds of rechargeable metallic lithium batteries, it is more complicated to stabilize a metallic lithium anode in a Li–S battery owing to double damage from dendrite formation and the side reaction between lithium polysulphide and metallic lithium during cycling. From the scanning electron microscopy (SEM) images shown in Fig. 5a–d , it is obvious that SIS-7# shows the lowest roughness and damage level of metallic lithium anode compared with the other three samples (2#: Fig. 5b , 4#: Fig. 5c and SIS-7#: Fig. 5d ), which demonstrates that the SIS electrolyte system can effectively reduce the corrosion and suppress the formation of lithium dendrites owing to the ultrahigh lithium salt concentration and high viscosity. It is generally accepted that dendrites start to grow in the non-aqueous liquid electrolyte when the anion is depleted in the vicinity of the electrode where plating occurs according to Chazalviel model [50] , [51] . In the case of SIS electrolyte with ultrahigh salt concentration, there is a mass of anion to keep the balance of cation (Li + ) and anion (TFSI − ) near metallic lithium anode, and the space charge that is created by TFSI − depletion is minimal, thus this is not a favourable condition for dendrite growth. Furthermore, owing to both ultrahigh lithium salt concentration and high lithium-ion transference number (0.73), SIS electrolyte provides a large amount of available lithium-ion flux and raises the lithium ionic mass transfer rate between electrolyte and metallic lithium electrode, thereby enhancing the uniformity of lithium deposition and dissolution in charge/discharge process. Besides, influenced by high viscosity, on the one hand, it possibly increases the pressure from the electrolyte to push back growing dendrites, resulting in a more uniform deposition on the surface of the anode. On the other hand, high viscosity limits anion convection near deposition area, which is also helpful to deposit uniformly [52] . 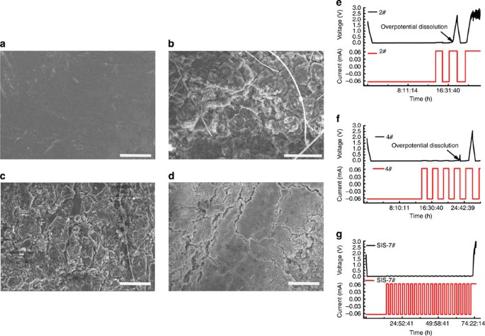Figure 5: Typical scanning electron microscopy images of metallic lithium anodes and lithium deposition and dissolution experiments. (a) Fresh lithium metal, (b) Lithium metal with 2# electrolyte after 278 cycles. (c) Lithium metal with 4# electrolyte after 183 cycles. (d) Lithium metal with SIS-7# electrolyte after 280 cycles. The white scale bar represents 60 μm for all the images; lithium deposition and dissolution experiments by electrochemically depositing Li on Cu foil (Current: 0.1 mA cm−2; the first deposition: 5 C cm−2; cycling process: 10% depth of discharge and 20 cycles; final dissolution: charged to 3 V). (e) 2# electrolyte. (f) 4# electrolyte. (g) SIS-7# electrolyte. The lithium cycling efficiency is calculated according to Aurbachet al.53 Figure 5: Typical scanning electron microscopy images of metallic lithium anodes and lithium deposition and dissolution experiments. ( a ) Fresh lithium metal, ( b ) Lithium metal with 2# electrolyte after 278 cycles. ( c ) Lithium metal with 4# electrolyte after 183 cycles. ( d ) Lithium metal with SIS-7# electrolyte after 280 cycles. The white scale bar represents 60 μm for all the images; lithium deposition and dissolution experiments by electrochemically depositing Li on Cu foil (Current: 0.1 mA cm −2 ; the first deposition: 5 C cm −2 ; cycling process: 10% depth of discharge and 20 cycles; final dissolution: charged to 3 V). ( e ) 2# electrolyte. ( f ) 4# electrolyte. ( g ) SIS-7# electrolyte. The lithium cycling efficiency is calculated according to Aurbach et al . [53] Full size image Meanwhile, lithium cycling efficiencies in different electrolyte systems were investigated by means of a Li deposition-dissolution experiment according to Aurbach et al . [53] (2#: Fig. 5e , 4#: Fig. 5f and SIS-7#: Fig. 5g ). In the commonly used low-salt concentration electrolyte system, the lithium cycling efficiency is estimated to be below 50%, which means a large excess of lithium as an anode needed in a real battery, thus decreasing the energy density and increasing the cost. In contrast, interestingly, a lithium cycling efficiency as high as 71.4% is obtained in the SIS-7# electrolyte system, which is much higher than that of other LiTFSI-based non-aqueous electrolytes [54] . Furthermore, from SEM images ( Supplementary Fig. S9 ), a smoother and more uniform lithium deposition was also clearly observed in the SIS-7# electrolyte system. This important issue for real applications has seldom been discussed in previous work on Li–S batteries. The different lithium cycling efficiencies in different electrolyte systems could be ascribed to the nature of solid electrolyte interphase (SEI) formed on the surface of lithium electrodes. To confirm our conjecture, X-ray photoelectron spectroscopy analysis of Li electrode surfaces was performed. Based on the previous work from Aurbach group [53] , [54] , [55] , [56] , [57] and our experimental data, it could be concluded that the solvents of DME and DOL in electrolytes could possibly be reduced to ROLi species and oligomers with −OLi end group, and the salt of LiTFSI could possibly be reduced to Li 3 N, LiF, C 2 F x Li y and sulphur-containing compounds such as Li 2 S, Li 2 S 2 O 4 , Li 2 SO 3 or SO 2 CF x during the cycling process to form an SEI layer on the metallic lithium surface ( Supplementary Fig. S10 ). The composition of SEI for both 2# and SIS-7# electrolytes seems to be similar; however, the thickness is different. In the case of SIS-7# electrolyte, it can be seen that the lithium metal signal appears after 150 s sputtering with Ar + ions, which etches the surface layer-by-layer from a lithium electrode. However, the signal still does not show up after 800 s sputtering for the lithium electrode cycled in the low-salt concentration electrolyte ( Fig. 6 ). This indicates that the thickness is different in these two electrolyte systems. 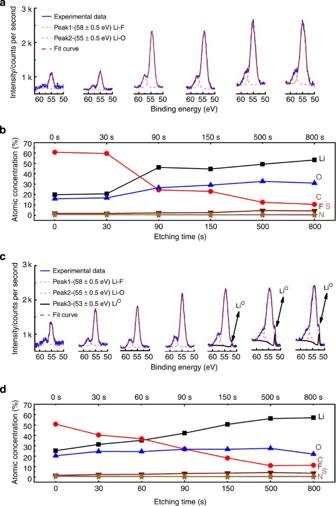Figure 6: X-ray photoelectron spectroscopy (XPS) analysis of metallic lithium anodes. After 100 cycles at a current rate of 0.2C with 2# and SIS-7# electrolytes, (a) XPS Li1sspectra of metallic lithium electrode using 2# electrolyte before sputtering and after sputtering with different times. (b) Summary of the atomic concentration of Li, C, O, S, N and F on the Li anode surface as a function of sputtering time using 2# electrolyte. (c) XPS Li1sspectra of metallic lithium electrode using SIS-7# electrolyte before sputtering and after sputtering with different times. (d) Summary of the atomic concentration of Li, C, O, S, N and F on the Li anode surface as a function of sputtering time using SIS-7# electrolyte. Figure 6: X-ray photoelectron spectroscopy (XPS) analysis of metallic lithium anodes. After 100 cycles at a current rate of 0.2C with 2# and SIS-7# electrolytes, ( a ) XPS Li 1 s spectra of metallic lithium electrode using 2# electrolyte before sputtering and after sputtering with different times. ( b ) Summary of the atomic concentration of Li, C, O, S, N and F on the Li anode surface as a function of sputtering time using 2# electrolyte. ( c ) XPS Li 1 s spectra of metallic lithium electrode using SIS-7# electrolyte before sputtering and after sputtering with different times. ( d ) Summary of the atomic concentration of Li, C, O, S, N and F on the Li anode surface as a function of sputtering time using SIS-7# electrolyte. Full size image In summary, we propose a new class of SIS electrolyte for the next-generation high-energy rechargeable metallic lithium batteries and take the electrolyte system of LiTFSI and ether solvents as an example to demonstrate the power of SIS electrolyte. For the appealing application in Li–S batteries, it is demonstrated that SIS electrolytes can not only inhibit the dissolution of lithium polysulphide but also effectively protect a metallic lithium anode against the formation of lithium dendrites, which makes the cell exhibit both excellent electrochemical performance and high safety. As a matter of fact, we anticipate further conceptual design of other SIS electrolyte systems by selecting appropriate salt and solvent components and adjusting these proportions according to different requirements for different rechargeable metallic lithium batteries (for example Li-O 2 batteries). It is expected that this class of SIS electrolyte would offer a new and important approach for improving the electrochemical and safety performance for metallic lithium batteries and further make us reconsider them without their past safety concerns. Synthesis The SIS electrolytes are prepared as follows: lithium bis(trifluoromethane sulphonyl) imide (LiN(SO 2 CF 3 ) 2 , LiTFSI) (TCI, Japan) and purified DME:DOL=1:1 by volume (Ferro, Suzhou, China) were mixed by ratio of mole number to volume, which are 1#: 1 mol per l, 2#: 2 mol per l, 3#: 3 mol per l, 4#: 4 mol per l, SIS-5#: 5 mol per l, SIS-6#: 6 mol per l and SIS-7#: 7 mol per l, respectively. The mixtures were stirred for 24 h at room temperature. All the experiments were performed in an argon-filled glove box. The carbon/sulphur composite is prepared by a melt-diffusion method. According to Ji et al . [10] , CMK-3 (Nanjing XF-nano, China) or Ketjenblack and sulphur were ground together, sealed in a glass tube containing argon, and heated at 155 °C for 24 h. (see Supplementary Figs S11–S13 and Supplementary Table S3 ). Characterizations The conductivity of electrolyte system was measured with an impedance analyser (Zahner Zennium, Germany) over a temperature range of −20 to 60 °C in a thermostated container. The lithium-ion transference numbers were obtained by combining alternating-current (AC) impedance and direct-current (DC) polarization measurements using a symmetric Li/electrolyte/Li cell. First, AC impedance test was performed to obtain a total resistance R cell . Then DC polarization was carried out to obtain a stable current I DC . The lithium-ion transference number was calculated by the formulas ( t Li+ = R cell / R DC and R DC = V DC / I DC ). DSC measurements were performed with a NETZSCH DSC 200F3 by sealing ~10 mg of the sample in an aluminium pan. The pan and the electrolyte were first cooled to about −150 °C with liquid nitrogen and then heated to 50 °C at a heating rate of 10 °C min −1 under nitrogen flow. The viscosity (η) of the electrolytes was measured on a programmable viscometer (Brookfield, DV-iii+) at 25 °C in a homemade dry chamber (H 2 O <10 p.p.m. ), and the temperature was accurately controlled to within ±0.1 °C using a Brookfield TC-502 oil bath. A SEM microscopy (Hitachi S-4800) equipped with a vacuum transfer box was used to study the morphology of the samples. The samples of lithium metal anode were stored in vacuum transfer box in an argon-filled glove box and transferred into SEM chamber without exposure to air. X-ray photoelectron spectroscopy analyses were performed in ESCALAB 250 using a monochromatized Al Kα source and equipped with an Ar + ion sputtering gun (Thermo Fisher). Ar + etching was conducted at an argon partial pressure of 10 −8 Torr in the x – y scan mode at ion acceleration of 3 kV and ion beam current density of 1 μA mm −2 . The lithium polysulphide dissolution experiments were carried out in the following: Li 2 S and S with a mole ratio of 1:7 (49.5 and 224 mg) were mixed and added in 2-ml pure solvent, 2 mol salt per 1-l solvent (2#), 4 mol salt per 1-l solvent (4#) and 7 mol salt per 1-l solvent (SIS-7#), respectively. The colour changes of solutions with time were observed and recorded by digital camera. The samples of 2#, 4# and SIS-7# after standing for 18 days were diluted with the corresponding electrolytes in the ratio of 1:7 for UV-Vis measurement, which was carried out on a Cary 5000 UV-Vis spectrophotometry (Varian, America). The control samples are pure electrolytes without Li 2 S 8 (4#′ and SIS-7#′). X-ray powder diffraction analysis was characterized by X’Pert Pro MPD X-ray diffractometer (Philips, Holland) using Cu–Ka radiation (1.5405 Å). Electrochemistry The electrode was fabricated by mixing C/S composite, carbon nanotube, poly(vinylidene difluoride) in weight ratio of 8:1:1 for cycle life measurement and the other weight ratio of 7:2:1 for rate capability measurement. The slurry was cast on carbon-coated Al current collector and dried at 50 °C in vacuum for 10 h. The coin cells CR2032 were assembled with the electrode, pure lithium foil as counter electrode and a glass fibre separator in an argon-filled glove box. The discharge and charge measurements at room temperature and low-temperature range of −20 to 0 °C in a thermostated container were carried out on a Land BT2000 Battery Test System (Wuhan, China). The average cycling efficiency of metallic lithium electrodes in various electrolytes (2#, 4#, SIS-7#) was performed by electrochemically depositing Li on Cu foil (5 C cm −2 ) followed by Li stripping and deposition cycling (10% depth of discharge-DOD, 0.1 mA cm −2 , 20 cycles). The residual Li was then dissolved electrochemically (charged to 3 V) on a Land BT2000 Battery Test System. The average Li cycling efficiency was calculated according to Aurbach et al . [53] How to cite this article: Suo, L. et al . A new class of Solvent-in-Salt electrolyte for high-energy rechargeable metallic lithium batteries. Nat. Commun. 4:1481 doi: 10.1038/ncomms2513 (2013).